Real-time influenza forecasts during the 2012–2013 season Recently, we developed a seasonal influenza prediction system that uses an advanced data assimilation technique and real-time estimates of influenza incidence to optimize and initialize a population-based mathematical model of influenza transmission dynamics. This system was used to generate and evaluate retrospective forecasts of influenza peak timing in New York City. Here we present weekly forecasts of seasonal influenza developed and run in real time for 108 cities in the USA during the recent 2012–2013 season. Reliable ensemble forecasts of influenza outbreak peak timing with leads of up to 9 weeks were produced. Forecast accuracy increased as the season progressed, and the forecasts significantly outperformed alternate, analogue prediction methods. By week 52, prior to peak for the majority of cities, 63% of all ensemble forecasts were accurate. To our knowledge, this is the first time predictions of seasonal influenza have been made in real time and with demonstrated accuracy. Influenza is associated with the deaths of 3,000–49,000 people each year in the USA [1] and presents an enormous burden on worldwide public health [2] . In temperate regions, pronounced outbreaks of influenza typically occur during winter. This recognized timing allows public health agencies to organize their influenza-related mitigation and response activities in preparation for the winter influenza season. For example, vaccines can be administered each fall in advance of expected increased winter incidence, and influenza antivirals can be stockpiled to meet high wintertime demand. While the general wintertime peak of influenza incidence in temperate regions is well described and predictable, the specific timing, magnitude and duration of individual local outbreaks in any given year are highly variable. Even after an outbreak has begun, it remains difficult to predict the future characteristics of the epidemic curve. If those outbreak characteristics were to be reliably forecast, public health response efforts could be better coordinated. Indeed, accurate forecast of the intensity and timing of infectious disease outbreaks discriminated among cities or regions within a country would provide greater lead time for preferential focus of mitigation and response resources to areas with more urgent need. In a recent study we showed that accurate and reliable predictions of seasonal influenza outbreaks can be made using a mathematical model representing population-level influenza transmission dynamics, which has been recursively optimized using an ensemble data assimilation technique and real-time estimates of influenza incidence [3] . This initial influenza forecast system was constructed and validated with a simple susceptible-infected-recovered-susceptible (SIRS) model [4] . In addition to the intrinsic effects of population level susceptibility on influenza transmission rates, influenza transmission in the model population is also modulated by observed daily absolute humidity (AH) conditions, as this meteorological condition has been shown to affect the survival and transmission of influenza [5] . Most relevant to this application, the SIRS model simulates the number of people in a local population infected with influenza at any point in time over the course of an outbreak. The SIRS model is described by two coupled equations, consisting of model state variables and parameters (See Methods). As the model is integrated forward in time, the state variables represent the number of infected and susceptible people within the simulated population. Model parameters describe additional intrinsic characteristics of both the host population and the virus. To perform a forecast, a 200-member ensemble of SIRS model simulations is numerically integrated for a given location (for example, New York City) and influenza season. Each ensemble simulation is initialized with a different randomly drawn suite of SIRS model state variables and parameters. Weekly local estimates of influenza incidence are then assimilated into these simulations using a data assimilation technique called the ensemble adjustment Kalman filter (EAKF) [6] . The EAKF is used to iteratively adjust both observable and unobservable state variables (that is, the number of newly infected and susceptible people, respectively), as well as the parameters of the SIRS model. These adjustments not only directly modify model estimates of infected and susceptible people in the simulated population, but also improve the ability of the model to replicate the future unfolding trajectory of a local outbreak by adjusting the model parameters. Parameter estimation is an important feature of the forecast system, as it allows the SIRS model to flexibly simulate outbreaks with very different characteristics. The process of informing the model with observations can be thought of as a ‘training’ period prior to an actual forecast. The assimilation of observations up to the time of forecast essentially optimizes the future behaviour of the ensemble to better match the evolving dynamics of the local seasonal outbreak. Actual weekly forecasts are then generated by integrating the ensemble of simulations into the future beyond the latest observation. A variety of quantities describing the epidemic curve can be forecast and evaluated (for example, peak timing, total outbreak cases). In prior work, we focused on the prediction of peak timing. For retrospective forecasts generated for New York City, we found a relationship between the spread of ensemble predictions of this metric and the accuracy of those predictions [3] . Indeed, forecast accuracy tended to improve as the spread of the ensemble decreased. The strength of this relationship is an important outcome, as it suggests that confidence in a particular forecast is inferable from the forecast ensemble variance. Those previous forecasts for New York City were generated using the humidity-forced SIRS model, Google Flu Trends (GFT) estimates of influenza-like illness (ILI) [7] , [8] and the EAKF. Here we present real-time forecasts of influenza incidence throughout the USA generated for the 2012–2013 season using a similar prediction system, but with a modified observational estimate of influenza incidence. Recent analysis indicates that scaling an ILI metric by the proportion of ILI patients testing positive for influenza can provide a more specific metric of influenza activity than ILI alone [9] . In near-real time, weekly estimates of the influenza-positive proportion of patients presenting with ILI are available for the USA by region [10] . For this work, we use such a combined metric, termed ILI+, in which municipal weekly GFT ILI estimates are multiplied by US Centers for Disease Control and Prevention (CDC) census division influenza positive proportions (see Methods). Indeed, ILI+ outbreaks tend to begin later in the season than ILI, which contains early fall signal that often reflects outbreaks of other respiratory infectious agents such as rhinovirus, rather than influenza activity [11] . Using the SIRS-EAKF framework and ILI+ observations, weekly real-time ensemble predictions of influenza epidemic progression were made for 108 cities throughout the USA during the 2012–2013 season. Here we show that these real-time forecasts accurately predicted local outbreak peaks up to 9 weeks in advance and that the expected accuracy of these ensemble predictions was inferable from the spread of the ensemble. Furthermore, we show that the SIRS-EAKF forecasts were substantially more accurate than alternate, analogue predictions. The findings indicate that accurate, calibrated real-time forecast of influenza outcomes can be generated with a simple dynamical model that has been optimized using real-time observations of influenza incidence and data assimilation methods. Retrospective calibration of 2012–2013 predictions Our calibration of the real-time influenza predictions over the USA during the 2012–2013 season is based on retrospective forecasts for the 2003–2004 through 2011–2012 seasons for 115 cities in the USA (see Methods). All retrospective ensemble simulations were trained each week to the point of forecast using scaled ILI+ observations and the EAKF. The 2008–2009 and 2009–2010 seasons, which included pandemic H1N1 outbreaks, were omitted from the analysis to restrict focus to the prediction of seasonal influenza. An analysis of peak timing forecast performance was carried out for all municipalities within a census division region, all cities in aggregate and individual municipalities ( Fig. 1 and Supplementary Fig. S1 ). Forecasts for which the ensemble predicted mode outbreak peak is 1–3 and 4–6 weeks in the future show a strong relationship of increasing accuracy with decreasing ensemble spread in most regions. This relationship allows us to quantify the expected accuracy of a predicted outcome based on the variance of the forecast ensemble. Only the New England census division, which contains only 3 of the 115 retrospective forecast cities, has no relationship at either of these lead times. The 7–9 week and 10+ week lead forecasts do not show a consistent relationship between spread and accuracy; however, the Mid-Atlantic, South Atlantic, East North Central and West North Central census divisions exhibit increasing forecast accuracy with decreasing ensemble spread. 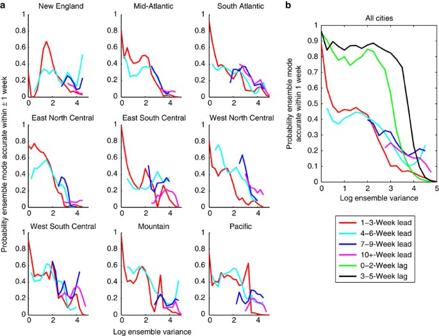Figure 1: Calibration of forecast accuracy as a function of ensemble spread. Retrospective forecasts of outbreak peak timing initiated for each of the 2003–2004 through 2011–2012 seasons, excluding the pandemic seasons of 2008–2009 and 2009–2010. Retrospective forecasts were made for 115 cities, which were then aggregated by census division or nationally. Plots present the probability that an ensemble predicted mode peak timing is accurate within ±1 week of the observed ILI+ peak as a function of ensemble predicted peak timing variance log transformed. (a) Training and forecast made using climatological AH, census division aggregation; (b) as in (a), but aggregated nationally. The coloured lines are for ensemble mode peak predictions 10+ weeks in the future (magenta), 7–9 weeks in the future (blue), 4–6 weeks in the future (cyan), 1–3 weeks in the future (red), 0–2 weeks in the past (green) and 3–5 weeks in the past (black). Figure 1: Calibration of forecast accuracy as a function of ensemble spread. Retrospective forecasts of outbreak peak timing initiated for each of the 2003–2004 through 2011–2012 seasons, excluding the pandemic seasons of 2008–2009 and 2009–2010. Retrospective forecasts were made for 115 cities, which were then aggregated by census division or nationally. Plots present the probability that an ensemble predicted mode peak timing is accurate within ±1 week of the observed ILI+ peak as a function of ensemble predicted peak timing variance log transformed. ( a ) Training and forecast made using climatological AH, census division aggregation; ( b ) as in ( a ), but aggregated nationally. The coloured lines are for ensemble mode peak predictions 10+ weeks in the future (magenta), 7–9 weeks in the future (blue), 4–6 weeks in the future (cyan), 1–3 weeks in the future (red), 0–2 weeks in the past (green) and 3–5 weeks in the past (black). Full size image When the retrospective forecasts are aggregated for all 115 cities, a smoother relationship emerges ( Fig. 1b ). Lead forecasts all exhibit increasing accuracy with decreasing ensemble variance, and forecasts for which the peak is predicted to have already occurred are accurate over a broad range of ensemble variances. Again, the emergence of a relationship between ensemble variance and forecast accuracy in the retrospective forecasts provides critical information for the interpretation of real-time forecasts and establishes a basis for determining whether the prediction system is well calibrated. If well calibrated, future events would occur in reality with the same probability as forecast by the system. Examination of the retrospective forecasts of peak timing for select major cities reveals considerable variability. Chicago is characterized by a strong relationship between prediction accuracy and ensemble variance at all forecast lead times, whereas Seattle is not ( Supplementary Fig. S1 ). New York City, which previously demonstrated a similar relationship of increasing prediction accuracy with decreasing ensemble variance for retrospective forecasts using GFT ILI estimates only [3] , here, when using ILI+ with the scaling used in this study (see Methods), does not exhibit this same relationship; however, at the Mid-Atlantic census division level such a relationship is broadly evident. Whether this variability among cities is a function of the limited number of years, the data type, the appropriateness of the model form, the scaling of the ILI+ estimates or the assimilation method is not currently understood. Ongoing evaluation of these issues will take place as the system is further developed. In the present, as the spatial scale at which information should be aggregated is to be yet determined, we present forecast results at municipal, regional and national scales. Forecast accuracy during the 2012–2013 season During the 2012–2013 USA influenza season, ILI+ observations and the EAKF were used to train the SIRS model, which was then used to create local near real-time forecasts of influenza activity for 108 municipalities ( Supplementary Table S1 ). Forecasts were generated each week upon release of the latest CDC census division influenza positive proportions. New CDC weekly data were initially released 6 days following the end of the most recently completed week (that is, near real time), and forecasts were produced the same day. For example, the week 51 forecasts were produced on 28 December 2012, included assimilation of week 51 ILI+ estimates (that is, through 22 December 2012), and were run in forecast mode from 23 December 2012 onward. A 1-week lead prediction for this forecast implies predicted local influenza incidence peak during week 52 (23–29 December 2012). The accuracy of weekly ensemble mode predictions generated for individual cities was mixed ( Table 1 and Supplementary Table S2 ). Some municipalities, for example, Birmingham, AL, Kansas City, MO, Buffalo, NY, were accurately forecast throughout the influenza season, both before and after the observed local peak had passed. Outbreak peaks in other cities, such as Phoenix, AZ, Chicago, IL and New Orleans, LA, were never well predicted. Many cities showed increasing accuracy of prediction as the season progressed, for example, San Diego, CA, Atlanta, GA and Boston, MA. Overall forecast accuracy increased from 19 to 74% as the season progressed and more observations were entrained into the evolving model ( Table 1 and Supplementary Table S2 ). By week 52, 63% of all ensemble forecasts of mode peak week were accurate within 1 week. Table 1 Accuracy of weekly municipal forecasts. Full size table The accuracy of these forecasts far exceeded the accuracy of predictions derived from the resampling of historical outcomes, including conditional resampling constrained by the current state ( Fig. 2 , Supplementary Methods , Supplementary Table S3 ). By week 49, all weekly SIRS-EAKF predictions were significantly more accurate than these resampled predictions. At week 52, the SIRS-EAKF forecasts produced nearly twice as many accurate predictions as the best resampled forecast. In addition, the 2012–2013 real-time SIRS-EAKF forecasts accurately discriminated peak timing among the 108 cities forecast ( Supplementary Methods , Supplementary Fig. S2 ). That is, repeated random comparison of each city’s forecast with observations from a different city proved less accurate than with observations from the same city. SIRS-EAKF forecast discrimination of peak timing among cities was statistically significant ( P <0.05, based on bootstrapped confidence intervals) from week 50 onward. 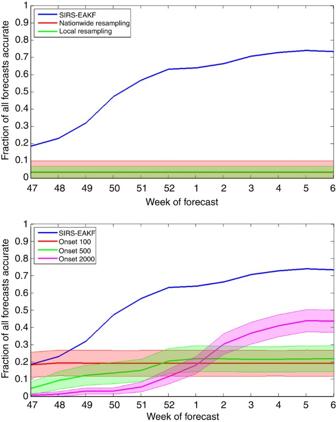Figure 2: Accuracy of 2012–2013 real-time forecasts. Plots comparing the weekly fraction of accurate SIRS-EAKF forecasts with the accuracy of analogue forecasts derived from historical probabilities (seeSupplementary Methods). Top: weekly SIRS-EAKF forecast accuracy and resampled predictions using two alternate resampling approaches. Bottom: weekly SIRS-EAKF forecast accuracy and resampled analogue predictions based on historically observed durations between initially elevated ILI+ and peak ILI+. Only cities that have exceeded an onset, or initial threshold, level of elevated ILI+ are included in the analogue forecast for a given week. Three different onset thresholds are shown as follows: 100, 500 and 2,000 ILI+. For all the analogue forecasts, the thick line depicts the mean fraction of accurate forecasts while the shading and thin lines delineate 95% bootstrap confidence intervals. Figure 2: Accuracy of 2012–2013 real-time forecasts. Plots comparing the weekly fraction of accurate SIRS-EAKF forecasts with the accuracy of analogue forecasts derived from historical probabilities (see Supplementary Methods ). Top: weekly SIRS-EAKF forecast accuracy and resampled predictions using two alternate resampling approaches. Bottom: weekly SIRS-EAKF forecast accuracy and resampled analogue predictions based on historically observed durations between initially elevated ILI+ and peak ILI+. Only cities that have exceeded an onset, or initial threshold, level of elevated ILI+ are included in the analogue forecast for a given week. Three different onset thresholds are shown as follows: 100, 500 and 2,000 ILI+. For all the analogue forecasts, the thick line depicts the mean fraction of accurate forecasts while the shading and thin lines delineate 95% bootstrap confidence intervals. Full size image Expected forecast accuracy for the 2012–2013 season The preceding validations demonstrate that the 2012–2013 predictions greatly outperformed predictions derived from historically inferred probabilities. However, these comparisons treat all SIRS-EAKF ensemble predictions as equal, when in fact each real-time ensemble prediction has an associated expected accuracy (for example, a 70% probability that influenza will peak in 5 weeks), which is inferred from the ensemble distribution of predicted outcomes ( Supplementary Fig. S3 ) and retrospective prediction accuracy ( Fig. 1 and Supplementary Fig. S1 ). In general, predictions for which there is greater spread among ensemble members have a lower expected accuracy than those with narrower distributions. Depending on whether this inference is based on retrospective forecasts aggregated at the national, regional or municipal, the expected accuracy of each prediction varies. Results from near real-time forecasts made for the 2012–2013 US influenza season during week 47 of 2012 through week 8 of 2013 indicate that the forecasts across all 108 cities were reasonably well matched with retrospectively calibrated confidences at the national scale ( Fig. 3 ). Specifically, forecasts predicting a local outbreak peak in 4–6 weeks, match historically expected accuracies, that is, predictions of peak timing 5 weeks in the future with a log ensemble variance of 2, were accurate ~50% of the time, which is slightly better than historical expectance. Predictions with a 1–3-week lead were weaker than expected for log ensemble variances >1.5 and <0.25, but better than expected between 0.5 and 1.5. The 7–9 week lead predictions greatly outperformed historical expectance. 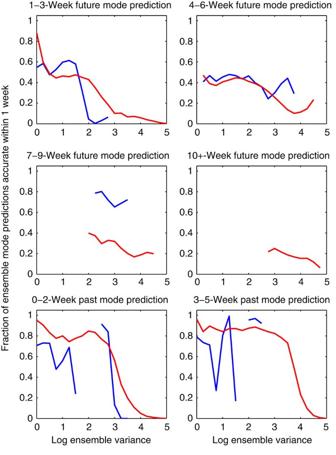Figure 3: Expected accuracy of peak timing forecasts for the 2012–2013 season. Week 47 (2012) through week 48 (2013) forecasts were made for 108 cities, which were then aggregated nationally. Plots present the probability that an ensemble predicted mode peak timing is accurate within ±1 week of the observed ILI+ peak as a function of ensemble predicted peak timing variance log transformed. The blue lines are the 2012–2013 predictions grouped by forecast lead; the red lines are the expected accuracy based on the retrospective forecasts also aggregated nationally (as shown inFig. 1b). Figure 3: Expected accuracy of peak timing forecasts for the 2012–2013 season. Week 47 (2012) through week 48 (2013) forecasts were made for 108 cities, which were then aggregated nationally. Plots present the probability that an ensemble predicted mode peak timing is accurate within ±1 week of the observed ILI+ peak as a function of ensemble predicted peak timing variance log transformed. The blue lines are the 2012–2013 predictions grouped by forecast lead; the red lines are the expected accuracy based on the retrospective forecasts also aggregated nationally (as shown in Fig. 1b ). Full size image On the other hand, predictions that the peak had passed mostly underperformed nationally scaled expectance. Too many forecasts were generated indicating the peak had passed only to witness observed ILI+ continue to rise. We believe this underperformance stems in part from the intense media attention accorded the influenza outbreak during 2012–2013 in the USA, which seems to have inflated GFT ILI estimates during January and prolonged a number of local outbreaks that in reality likely peaked in late December [12] . When the predictions are grouped by census division region and compared by lead time and ensemble spread to expected accuracies the results are more mixed ( Supplementary Fig. S4 ). The accuracy of 2012–2013 predictions was similar to regional historical expectance for some lead times and regions, for example, the West South Central, Mountain and Pacific census division regions with a 4–6 week lead, but most other groupings diverged from expectance. Similar examination of individual city forecast accuracy versus expected accuracy reveals very mixed results ( Supplementary Fig. S5 ). The 1–3 week lead predictions for Chicago, Dallas, Houston, Memphis and St Louis were not accurate, nor in line with accuracy as expected at the municipal, regional or national scale. Conversely, the 1–3 week peak timing predictions for Los Angeles, San Francisco, and Seattle outperformed municipal, regional and national expected accuracies at low ensemble spread, for Miami outperformed regional and national expected accuracies at all ensemble spreads, and for New York City outperformed all expected accuracies for all ensemble spreads. Clearly, the New York City municipally calibrated accuracy, which performed poorly in retrospective prediction ( Supplementary Fig. S1 ), did not provide a reliable estimate of forecast accuracy expectance during 2012–2013. These findings indicate that nationally aggregate retrospective forecast accuracy provided a better estimate of expected accuracy of the real-time forecasts across the USA than regional and municipal expected accuracies. We can thus use real-time forecast ensemble variance to discriminate more reliable municipal predictions (for example, 90% expected accuracy) from less reliable municipal predictions (for example, 20% expected accuracy) using nationally aggregated expected accuracy. Challenges due to elevated ILI+ levels during 2012–2013 During the 2012–2013 US influenza season, ILI+ in most of the 108 forecast cities peaked during weeks 2–4 ( Supplementary Fig. S6 ). These late-peaking cities, perhaps due to a longer period for ILI+ training prior to the peak, tended to be better predicted than cities that peaked earlier ( Supplementary Fig. S6B , Supplementary Table S4 ). A number of the cities that were forecast poorly had observed, seasonal cumulative ILI+ that, when scaled to reflect the total number of people infected within the SIRS model, neared or even exceeded the total population ( Supplementary Fig. S7 ). Indeed, with the scaling presented here ( γ =2.5, see Methods), 17 of the 108 forecast cities experienced total ILI+, that is, week 40 (2012) to week 12 (2013) summed weekly incidence, in excess of the model population ( N =100,000). These aggregate incidence levels were unprecedented. During the seven retrospectively forecast seasons, across all cities and with identical γ scaling, seasonal total ILI+ never exceeded 70,000, whereas during 2012–2013, 60 of 108 cities exceeded this threshold. The 2012–2013 elevated ILI+ levels were a product of bias in GFT ILI relative to CDC ILI, possibly brought about by intense media coverage of the USA influenza outbreak, as well as the virulence of some of the circulating influenza strains, which likely prompted a higher percentage of infected persons to seek medical attention than in most previous years [12] (see Methods). Even with continual state variable and parameter adjustment via the EAKF, the SIRS model, as formulated for a single influenza strain, is not equipped to depict an outbreak near or in excess of its total population ( Supplementary Fig. S8 ). Indeed, 2012–2013 real-time forecast accuracy was negatively correlated with seasonal total ILI+ (for example, correlation of week 1 municipal forecast accuracy with seasonal total ILI+: r =−0.30, P =0.0019, two-sided t -test). These findings suggest that forecast accuracy during the 2012–2013 season was undermined by higher than normal values of scaled ILI+. Examination of forecast time series ( Supplementary Fig. S8 ) indicates that predictions for cities with high total ILI+ generally under-represented outbreak magnitude. While such performance is sub-optimal, it is encouraging as it suggests that peak timing forecast accuracy might have been still better in the absence of these unusual biases. Furthermore, a number of potential remedies exist for handling such biases in the future (see Supplementary Note 1 ). Sensitivity to different observational estimates of incidence During January of the 2012–2013 season, GFT ILI estimates considerably overestimated target CDC reported ILI [12] . As long as the same data source is used both to train and validate the SIRS-EAKF forecasts, and as long as within-season changes in data bias are not too extreme, the ensemble forecasts should perform well. However, due to the January increase of GFT ILI bias, the forecast validation metric, ILI+ peak timing, may not represent reality well. Obviously, to best inform public health, we would prefer an observational estimate of weekly influenza infections that represents actual incidence as accurately as possible. CDC ILI estimates are not made publicly available at the municipal scale; however, they are available in near real time at aggregate national and regional levels, and both GFT ILI and CDC ILI estimates are provided in near real time at the Health and Human Service (HHS) region scale. We therefore ran regional-scale comparison forecasts using HHS GFT ILI+ and HHS CDC ILI+ estimates (see Supplementary Methods ). Owing to the large geographic scale of each region, the SIRS model was run without AH-forced modulation of transmissibility; instead, R 0 was treated as a free parameter to be optimized by the EAKF assimilation process. HHS CDC ILI+ peaked during week 52 of the 2012–2013 season for all divisions except the HHS Region 9, which peaked during week 4 ( Fig. 4 ). In contrast HHS region GFT ILI+ estimates peaked during week 1 (HHS Region 5), week 2 (HHS Regions 1–4), week 3 (HHS Regions 6–8) and week 4 (HHS Regions 9–10). The weekly total accuracy of HHS-region CDC ILI+ forecasts ranged from a low of 59.5% (week 52) to a high of 90% (week 5). Overall, accuracy is greater for the HHS-region CDC ILI+ forecasts than the HHS-region GFT ILI+, which degraded in forecast quality as the season progressed from a high total accuracy of 85.2% (week 48) to a low of 46.7% (week 4). This degradation of HHS GFT ILI+ forecast accuracy coincides with the January increase of GFT ILI bias relative to CDC ILI. On average during weeks 1–5 of 2013, HHS-region GFT ILI+ was 2.20 times HHS-region CDC ILI+. 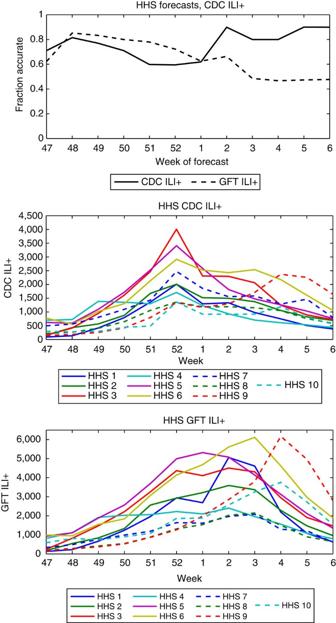Figure 4: Weekly predictions of CDC ILI+ and GFT ILI+ peak timing for HHS regions. Top: the fraction of all SIRS-EAKF forecasts each week (made using SIRS model without AH modulation ofR0); the week 1–6 forecasts were run in near real time; the week 47–52 forecasts were run using data downloaded following week 1. Middle: plots of observed HHS CDC ILI+ as reported through week 12, 2013; using this metric, all HHS peak during week 52, except HHS Region 9, which peaked during week 4. Bottom: plots of observed HHS GFT ILI+ as reported through week 12, 2013; 9 of the 10 GFT ILI+ HHS regions peak later than their counterpart CDC ILI+ estimate. From week 40 (2012) through week 12 (2013), HHS GFT ILI+ was on average 1.61 times corresponding estimates of HHS CDC ILI+, and during weeks 1–5 HHS GFT ILI+ was on average 2.20 times HHS CDC ILI+. Figure 4: Weekly predictions of CDC ILI+ and GFT ILI+ peak timing for HHS regions. Top: the fraction of all SIRS-EAKF forecasts each week (made using SIRS model without AH modulation of R 0 ); the week 1–6 forecasts were run in near real time; the week 47–52 forecasts were run using data downloaded following week 1. Middle: plots of observed HHS CDC ILI+ as reported through week 12, 2013; using this metric, all HHS peak during week 52, except HHS Region 9, which peaked during week 4. Bottom: plots of observed HHS GFT ILI+ as reported through week 12, 2013; 9 of the 10 GFT ILI+ HHS regions peak later than their counterpart CDC ILI+ estimate. From week 40 (2012) through week 12 (2013), HHS GFT ILI+ was on average 1.61 times corresponding estimates of HHS CDC ILI+, and during weeks 1–5 HHS GFT ILI+ was on average 2.20 times HHS CDC ILI+. Full size image While the HHS-region CDC ILI+ forecasts are more accurate, the HHS-region GFT ILI+ peak timing forecasts are still quite reliable. That is, real-time municipal GFT ILI+ forecast accuracy was not an artifact of GFT ILI biases (that is, even though the target is wrong, the SIRS-EAKF framework is trained for that target and predicts it well). The HHS findings also suggest that were CDC ILI estimates at the municipal scale available, our city forecasts ( Fig. 2 ) might have been more accurate. In addition, the results indicate that reliable influenza forecasts can be made without AH modulation of transmissibility. That is, local, non-linear transmission dynamics are more important for forecast accuracy than AH modulation of influenza transmissibility. A fuller exploration of these model design issues and the benefit of including AH in the SIRS model framework is forthcoming. This study has shown that forecast accuracy with the SIRS-EAKF system during the 2012–2013 influenza season was far superior to forecasts generated from resampling historically expected probabilities. This finding indicates that forecasting using a trained population-based influenza model that represents local non-linear transmission dynamics is much more informative than simple analogue expectance. This study has also shown that, when nationally aggregated, SIRS-EAKF ensemble forecast expected accuracy could be reliably inferred from the forecast ensemble spread. A further, more detailed exploration of the geographic variability of forecast accuracy and reliability is needed to determine whether some municipalities or regions are fundamentally more predictable. Preliminary analysis shows that for longer lead times (>2 weeks ahead of the observed ILI+ peak), municipal peak timing forecast accuracy increased as city population decreased, population density increased, or city area decreased ( Supplementary Table S5 , Supplementary Note 2 ). That is, longer lead forecasts for smaller populations, higher population densities or smaller geographies tended to be more accurate. This finding suggests that larger municipalities might be better forecast if broken into smaller geographic units. A fuller exploration of these issues is needed to verify this preliminary finding and to define the optimal spatial scales at which influenza should be forecast. In addition, the characteristics that make an influenza outbreak more or less predictable—including geographic area, population size and density, number of circulating strains, population age, duration of outbreak, number of peaks, and so on—need to be better identified. A more detailed evaluation of the timeliness and quality of real-time influenza incidence observation data forms is also needed. The latest ILI+ observations are first available 6 days following the conclusion of a given influenza week. This 6-day lag delays the production of new weekly predictions, which could be generated sooner if weekly estimates of influenza positive proportions [10] were reported more quickly. In addition, forecasts also might benefit from provision of these data at a finer spatial resolution (for example, municipal- or state level instead of regional level). Different forecast models also need to be tested. For example, during the 2012–2013 season in the USA, four strains of influenza (A/H3N2 Victoria/361/2011-like, B/Yamagata lineage, B/Victoria lineage and A/H1N1/California/7/2009-like) were in circulation. Our use of a single-strain SIRS model for the prediction of these multiple strain outbreaks is likely a source of bias that may have reduced the overall accuracy of the forecasts. Indeed, the SIRS-EAKF parameter estimates often appear slightly high ( Supplementary Fig. S9 , Supplementary Note 1 ), which indicates that the EAKF may be adjusting state variable and parameter estimates to compensate for model bias. In the future, we plan to develop and test forecasts using models that simulate individual influenza subtypes or strains. In addition, we also plan to investigate systematically how the form and structure of an outbreak influences its inherent predictability. Nevertheless, it is encouraging that a simple SIRS model, which neglects known aspects of influenza transmission, is already able to produce accurate, calibrated forecasts. During the 2012–2013 season, we trained and forecast each of the 108 forecast municipalities in isolation. In the future, alternate training and forecasting strategies might be adopted that account for the spatial co-variability of the parameters that control transmission dynamics or levels of modelled incidence and susceptibility. A number of other predictions should also be explored. Real-time forecast of additional outbreak metrics, such as attack rate and peak magnitude, needs to be assessed, and the model framework might be used to predict the timing of local outbreaks worldwide during pandemic events. Unlike attempts to describe the emergence of a pandemic strain [13] or the geographic spread of an emergent strain [14] , [15] , [16] , these efforts would be used to forecast the propagation of the pandemic strain through populations once local outbreaks have begun. Other pathogens such as rhinovirus or respiratory syncytial virus might also be forecast. In addition, prediction with alternate combinations of model form [17] , [18] , data type [10] , [11] and assimilation scheme [19] , [20] , [21] should be explored. Ultimately, an ensemble of different model forms, data types and assimilations each weighted by predictive ability in a given location may provide superior localized forecast of influenza activity. During the 2012–2013 influenza season, the real-time forecasts were archived for future study [12] and disseminated in real time on a weekly basis to officials at the CDC. At that time, these predictions were a novel, relatively untested data stream; it was thus not expected that officials would use the forecasts to inform their decisions. However, going forward, we must work with public health officials to increase their familiarity with the capabilities and limitations of these forecasts, as well as our own familiarity with the public health intervention and response decision-making process. By doing so, these forecasts can be more sensibly presented, interpreted and used in support of intervention and response decisions such as vaccine allocation, the distribution of anti-viral therapeutics and school closure. In the future, the real-time influenza forecasts will also be posted online. Different lead forecasts will likely have different practical uses for the broader public. Short-lead predictions (that is, 0–3 week leads) would likely improve awareness of current influenza risk, heighten vigilance to infection and increase attention to personal hygiene; long-lead predictions (that is, ≥5 weeks) would provide enough time for vaccine-induced generation of protective antibodies and thus may motivate more individuals to get vaccinated. In addition to this broader dissemination, an ongoing task will be to improve forecast accuracy and reliability. Just as the performance of weather forecasting systems has advanced over time, our hope is that the forecast of influenza and other seasonally recurring respiratory pathogens will also improve. Description of the SIRS model The model used for this study is a perfectly-mixed, absolute humidity-driven susceptible-infectious-recovered-susceptible (SIRS) construct [3] . This construct is a two-variable non-linear oscillator that describes the transmission of influenza within a local population. The SIRS model equations are: where S is the number of susceptible people in the population, t is time in years, N is the population size, I is the number of infectious people, N – S – I is the number of recovered individuals, β ( t ) is the contact rate at time t , L is the average duration of immunity, D is the mean infectious period and α is the rate of travel-related import of influenza virus into the model domain. The contact rate, β ( t ), is determined by , where R 0 ( t ), the basic reproductive number, is the number of secondary infections the average infectious person would produce in a fully susceptible population at time t. Absolute humidity (AH) modulates transmission rates within this model by altering R 0 ( t ) through an exponential relationship similar to how AH has been show to affect both influenza virus survival and transmission in laboratory experiments [4] : where R 0 min is the minimum daily basic reproductive number, R 0 max is the maximum daily basic reproductive number, a =180, and q(t) is the time-varying specific humidity, a measure of AH. The value of a is estimated from the laboratory regression of influenza virus survival upon AH [5] . As formulated above, this model contains two variables ( S and I ) and four parameters ( L, D, R 0 max and R 0 min ). S and I are continuous variables, such that fractional persons are simulated, which enables transitions between model states to be calculated directly from Equations 1 and 2 without any stochasticity. Simulations were performed with fixed travel-related seeding of 0.1 infections per day (1 infection every 10 days). Specific humidity data Specific humidity (SH) data were compiled from the National Land Data Assimilation System (NLDAS) project-2 data set. These data are derived through spatial interpolation, temporal disaggregation and vertical adjustment from station measurements and National Center for Environmental Prediction North American Regional Reanalysis [22] . The gridded NLDAS meteorological data are available in hourly time steps on a 0.125° regular grid from 1979 through the present [23] . Local SH data for each of the 115 cities included in these forecasts were assembled for 1979–2011. These hourly data were then averaged to daily resolution. A 1979–2002 (24-year) daily climatology was then constructed for each city and used as the daily specific humidity forcing for all retrospective forecasts. A 1979–2011 (33-year) daily climatology was constructed for each city and used for the real-time forecasts during the 2012–2013 influenza season. Observational estimates of influenza incidence GFT data [8] give estimates of weekly ILI per 100,000 people seeking medical attention based on a simple statistical model that uses internet search query activity as a predictor of US Centers for Disease Control and Prevention (CDC) ILI (see ref. 7 for details). GFT ILI data are available weekly in real time and, in the continental USA, provided at the municipal scale for 115 cities. Previously, we used GFT ILI as our estimate of respiratory infection incidence when retrospectively forecasting in New York City [3] . For this study, we employ an alternate metric that more precisely estimates influenza infection incidence. In the USA, CDC ILI is a measure of influenza among patients presenting at sentinel hospitals and clinics, which comprise the US Outpatient Influenza-like Illness Surveillance Network (ILINet). ILI is a symptomatic diagnosis requiring fever above 37.8 °C plus cough and/or sore throat. Patients for which the aetiology is known to be not influenza are not classified as ILI; however, the specific pathogen infecting most patients presenting with ILI is not typically determined. As such, the ILI designation includes patients with other respiratory viruses, such as rhinovirus and respiratory syncytial virus, who present with similar symptoms. Owing to this non-specificity, outbreaks of ILI tend to be of longer duration than pure influenza outbreaks. A cleaner signal of actual influenza infection incidence can be generated simply by multiplying ILI with a second observational estimate: the percentage of people presenting with ILI who tested positive for influenza (hereafter ‘influenza positive proportions’) [9] . Weekly US influenza positive proportions are compiled through the National Respiratory and Enteric Virus Surveillance System (NREVSS) and US-based World Health Organization (WHO) Collaborating Laboratories. The NREVSS and WHO laboratories assay volunteered respiratory swab samples from patients presenting with ILI for aetiological agents. The weekly data derived from this laboratory network provides an estimate of the percentage of patients presenting with ILI who are infected with influenza [10] . During the 2012–2013 influenza season these weekly data were first available with a lag, 6 days following the end of a given influenza week. In addition, unlike the GFT ILI estimates, which were available in real time at the municipal scale, influenza positive proportions were only available nationally and regionally. Still, by multiplying weekly municipal GFT ILI estimates by CDC census division regional influenza positive proportions for the same week, a near real-time estimate of municipal influenza infection per 100,000 patient visits can be made. Here we refer to this metric as ILI+ ( Supplementary Fig. S10 ). Outbreaks of ILI+ are of shorter duration than GFT ILI alone. In addition, observed ILI+ outbreak trajectories are more consistent with the transmission dynamics simulated within an influenza model. That is, model dynamics are more likely to produce an outbreak with the duration, peak magnitude and total number of cases seen in ILI+ than with ILI. Consequently, use of the ILI+ metric may provide a better observational target for a model simulating purely influenza transmission. In addition, the ILI+ target may also provide a better observation for recursive assimilation and optimization of the model, as well as forecast. In this study, 115 US cities were forecast retrospectively using the ILI+ observation metric and 108 US cities were forecast in near real time (6-day delay) during the 2012–2013 influenza season ( Supplementary Table S1 ). Nb: GFT stopped releasing ILI estimates for seven cities during the 2012–2013 influenza season, hence only 108 of the 115 cites were forecast in near real time. Scaling ILI+ to estimate influenza incidence To assimilate ILI+ observations into the SIRS model, these values must first be converted to influenza incidence, a variable that is distinct from I , but which can be tracked within the SIRS model. (incidence represents the number of new influenza infections during a week, whereas I is the number of infected persons at any point in time.) Conversion between ILI+ and influenza incidence is influenced by several factors. Specifically, ILI+ is simply an estimate of the probability for a given week that a person seeking medical treatment, m , has influenza, that is, . By Bayes theorem, ILI+ is then where p ( i ) is the probability of getting influenza in a given week (that is, influenza incidence), is the probability of seeking medical attention given infection with influenza, and p ( m ) is the probability that anyone seeks medical attention for any reason. Equation 4 can be rearranged as: where . That is, the probability of incident influenza infection in the general population, p ( i ), is approximately equal to ILI+ scaled by: 1 the probability that anyone seeks medical attention for any reason, p ( m ) 2 the probability that a person with influenza seeks medical attention, Both scaling probabilities change through time. In particular, changes with influenza virulence: an influenza strain producing more severe symptoms will increase the probability that an infected person seeks medical attention. We ran retrospective forecasts with , and found that values ranging from 2 to 15 had good predictive ability. For the 2012–2013 season, we generated weekly real-time forecasts using different values of between 2 and 15. As the season progressed, it became clear that one or more of the circulating influenza strains was highly virulent. As a consequence, we focused our forecasting efforts on lower scaling values, that is, . These are the forecasts presented in this paper (real-time forecasts made with alternate scaling factors, for example, , were archived and are available for analysis). In the future, the scaling factor, , might not be fixed but rather treated as a free parameter and adjusted during EAKF assimilation of observations. In the EAKF framework, the variance of observational error must be prescribed. For this work, we specified a heuristic observation error variance (OEV) that varied with the magnitude of the ILI+ estimate. Similar to Shaman and Karspeck [3] , the OEV for week k , was defined as where ILI+ j is the ILI+ estimate for week j. OEV has units of (infected people per 100,000 people) squared. Equation 6 indicates that there is a baseline uncertainty in estimates of influenza incidence that increases or decreases proportionally with ILI+ estimates summed for the preceding 3 weeks. Model training using EAKF Two hundred-member ensemble simulations with the SIRS model were trained up to the point of forecast using the scaled ILI+ observations and the EAKF. Throughout training, the EAKF algorithm updates the ensemble simulations of the observed state variable (that is, incidence) to better align with scaled ILI+ observations. Simultaneously, it uses cross ensemble co-variability to adjust both the unobserved state variables and parameters. In doing so, the ensemble simulations better match observed incidence levels and accrue other key variable and parameter characteristics needed to better mimic local outbreak dynamics. Unlike some Kalman filter forms that use random perturbations (that is, stochasticity) in conjunction with the Kalman gain to obtain each update, the EAKF algorithm uses a non-random, deterministic adjustment [6] , [24] . More details on the application of the EAKF to the SIRS are provided in the study by Shaman and Karspeck [3] . Multiplicative inflation was applied following the assimilation of each ILI+ observation of incidence [3] , [6] . The inflation was used to counter EAKF tendency towards ‘filter divergence', which occurs when the prior ensemble spread becomes spuriously small, causing the system to give too little weight to observations and to diverge from the true trajectory. For this application, the variance of the observed state variable, influenza incidence, was inflated by a multiplicative factor of λ =1.02 prior to each weekly observational assimilation and calculation of the posterior. The remaining model state variables and parameters were augmented with a 2% increase of all prior ensemble values. This augmentation increases the mean and variance of these model state variables and parameters prior to weekly assimilation of the observation and calculation of posterior values based on EAKF formulations and the co-variability of the observed state variable with model state variables and parameters. Retrospective forecasts Retrospective forecasts were performed using the humidity-forced SIRS model for the 2003–2004 through 2011–2012 influenza seasons. Influenza seasons begin around week 40 of the calendar year, corresponding to early October. This start date is typically before there is significant influenza activity. Focus is restricted to seasonal influenza prediction, so the 2008–2009 and 2009–2010 pandemic years were excluded from the analysis. For each year, assimilation of ILI+ data using a 200-member EAKF was initiated in the fall season with a random selection of initial state variables ( S and I ) and parameters ( L , D , R 0 max and R 0 min ). Each week the latest ILI+ observation was assimilated and a new posterior ensemble generated [6] . This posterior ensemble was then propagated forward to the next weekly observation and the assimilation process was repeated. At each week, forecasts were generated by integrating the model posterior forward without further training [3] to the end of the influenza season. To sample a more complete range of possible parameters and model states, the assimilation/forecast process outlined above was repeated 125 times. Specifically, 25 200-member ensembles were initialized with different randomly chosen initial parameters and state conditions and initiated at one of 5 staggered start weeks in the fall season (weeks 38, 39, 40, 41 or 42). Thus, for each of the 7 influenza seasons, 39 weekly retrospective forecasts were generated for each of 125 200-member ensemble simulations for each of 115 cities within the USA ( Supplementary Table S1 ). Initial state variable and parameter conditions for each ensemble member simulation were generated from the same prior for each of these ensemble simulations. The parameter ranges for this initial random selection were 2≤ L ≤10, 2≤ D ≤7, 1.3≤ R 0 max ≤4, 0.8≤ R 0 min ≤1.3, as in Shaman and Karspeck [3] , and combinations were selected using a Latin hypercube sampling strategy. By running multiple ensembles for each city, year and start date, the multiple forecasts generated provide a measure of variability of ensemble forecast statistics, that is how much the ensemble mode varies as a function of random initial conditions and start date. Analysis of retrospective forecasts The quality of the retrospective forecasts was analysed by comparing the accuracy of each ensemble mode prediction of peak timing with the spread of predictions among the 200 simulations within that ensemble [3] . A forecast is deemed accurate if the ensemble mode predicted peak lies within 1 week of the observed ILI+ peak. The spread is calculated as the log ensemble variance of the predicted peak weeks. Plots of mode accuracy versus ensemble spread indicate an inverse relationship in which the expected accuracy increases as the log ensemble variance decreases ( Fig. 1 and Supplementary Fig. S1 ). These relationships, stratified by lead of prediction provide an expectance of accuracy for the 2012–2013 real-time forecasts. Generation of real-time forecasts The 2012–2013 near real-time forecasts were generated using a broader range of start dates: weeks 32, 34, 36, 38, 40 and 42. For each of these six start dates, 25 200-member ensembles were initiated, each with a different suite of randomly chosen parameters and initial conditions. This is analogous to the procedure used to generate retrospective forecasts. Following assimilation of the most recent ILI+ observation and generation of a new posterior, the ensemble was integrated forward to the end of the season (a combined 40 weeks of training and forecast). Thus, for each city, 150 200-member ensemble forecasts were generated each week upon CDC release of the latest census division influenza positive proportions. This process created a distribution of 150 ensemble-mode peak timing predictions each week for each city (that is, each 200-member ensemble produces an ensemble mode prediction of peak timing). Often these 150 mode predictions were redundant, but in many instances, a range of mode predicted outcomes were realized (reflecting uncertainty in the ensemble forecasts). New influenza-positive proportions were initially released 6 days following the end of the most recently completed week. As a consequence, the forecasts were performed in ‘near real time’. For example, the week 52 forecasts were produced on 4 January 2013, the day the week 52 influenza positive proportions were released. These forecasts included assimilation of week 52 ILI+ estimates, and ran in forecast mode from 30 December 2012 onward. A 1-week lead prediction for this forecast implies predicted local influenza incidence peak during week 1 (30 December 2012 to 5 January 2013). The first forecast (week 47) was performed following assimilation of week 47 data. Results from forecasts generated for week 47 (2012) through week 8 (2013) are presented. How to cite this article: Shaman, J. et al. Real-time influenza forecasts during the 2012–2013 season. Nat. Commun. 4:2837 doi: 10.1038/ncomms3837 (2013). The content is solely the responsibility of the authors and does not necessarily represent the official views of the National Institute of General Medical Sciences, National Institutes of Health or Department of Homeland Security.